Fast sulfate formation from oxidation of SO2by NO2and HONO observed in Beijing haze Severe events of wintertime particulate air pollution in Beijing (winter haze) are associated with high relative humidity (RH) and fast production of particulate sulfate from the oxidation of sulfur dioxide (SO 2 ) emitted by coal combustion. There has been considerable debate regarding the mechanism for SO 2 oxidation. Here we show evidence from field observations of a haze event that rapid oxidation of SO 2 by nitrogen dioxide (NO 2 ) and nitrous acid (HONO) takes place, the latter producing nitrous oxide (N 2 O). Sulfate shifts to larger particle sizes during the event, indicative of fog/cloud processing. Fog and cloud readily form under winter haze conditions, leading to high liquid water contents with high pH (>5.5) from elevated ammonia. Such conditions enable fast aqueous-phase oxidation of SO 2 by NO 2 , producing HONO which can in turn oxidize SO 2 to yield N 2 O.This mechanism could provide an explanation for sulfate formation under some winter haze conditions. Beijing experiences severe air pollution events in winter, commonly called winter haze. The concentration of fine particulate matter with aerodynamic diameter less than or equal to 2.5 μm (PM 2.5 ) can exceed 200 μg m −3 on a 24-h average basis during these events [1] , considerably higher than the 24-h Chinese National Ambient Air Quality Standard of 75 μg m −3 . Winter haze events are often associated with high relative humidity (RH) [2] , [3] , [4] , [5] and a major contribution of sulfate to total PM 2.5 [6] . Sulfate is produced in the atmosphere by oxidation of sulfur dioxide (SO 2 ) emitted from coal combustion [7] , [8] . But the photochemical oxidants known to drive atmospheric oxidation of SO 2 (hydroxyl radical, hydrogen peroxide, ozone) have very low concentrations under typical winter haze conditions [7] , [9] , [10] . This has led to considerable debate regarding the mechanisms responsible for sulfate formation in winter haze [9] , [11] , [12] , [13] . The high-RH conditions characteristic of winter haze cause particulate matter to take up water, enabling aqueous-phase pathways for SO 2 oxidation. SO 2 is a weak acid with moderate water solubility (Henry’s law constant K H = 1.2 M atm −1 at 298 K) that dissociates in water to form bisulfite (HSO 3 − ; pK a,1 = 1.9 at 298 K) and sulfite (SO 3 2− ; pK a,2 = 7.2 at 298 K). Bisulfite and sulfite are converted to sulfate by a number of aqueous-phase oxidants with rates dependent on pH [14] . As the air cools at night or through rising motions the haze can turn to fog and low clouds (RH > 100%), increasing the atmospheric liquid water content (LWC) by orders of magnitude and hence the importance of SO 2 aqueous-phase oxidation pathways. Most previous studies of sulfate formation during Beijing haze events have focused on mechanisms taking place in the ubiquitous haze particles (RH < 100%) rather than in the more sporadic fog and cloud (RH > 100%) [13] , [15] , [16] , [17] . Haze particles are concentrated aqueous solutions with pH that can be estimated from standard thermodynamics [18] . Aqueous-phase oxidation of SO 2 by nitrogen dioxide (NO 2 ) in haze has been proposed [9] , [11] , [13] , with NO 2 originating from vehicular emissions, but requires higher pH than the 4–5 range inferred from thermodynamic calculations [19] , [20] , [21] . Some studies have suggested that oxidation by NO 2 would be enhanced by fog [9] , [13] , [17] . Aqueous-phase autoxidation of SO 2 by molecular oxygen catalyzed by transition metal ions (TMI) has been proposed [22] , [23] but is poorly constrained due to the lack of information on TMI concentration, complexation, and solubility [24] . A recent study suggests that aqueous-phase oxidation by hydrogen peroxide (H 2 O 2 ) in haze could be significant [10] . Yet another suggestion is that some of the reported sulfate could actually be hydroxymethanesulfonate (HMS) produced by in-cloud complexation of HSO 3 − and SO 3 2− with formaldehyde (HCHO) [25] , [26] . Here we present detailed chemical observations during a Beijing haze event in December 2016 where PM 2.5 concentrations reached 400 μg m −3 . We observe fast sulfate production as RH increases over the course of the event, leading to extensive nighttime fog and low clouds, and find a concurrent increase of nitrous oxide (N 2 O). N 2 O is a product of aqueous-phase SO 2 oxidation by dissolved nitrous acid (HONO) [27] , [28] , [29] , and observations of HONO during the event support this sulfate formation mechanism. Most of the HONO appears in turn to be produced by aqueous-phase SO 2 oxidation by NO 2 , leading us to propose a two-step fog-enabled mechanism for sulfate formation during winter haze events. 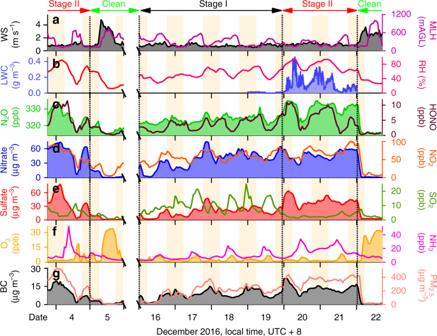Fig. 1: Chronology of a winter haze event. The figure shows the time series of meteorological parameters and chemical species measured in Beijing on December 4–22, 2016. The measurements were made from the roof of an Institute of Atmospheric Physics (IAP) building except for liquid water content (LWC) measured at the Beijing Observatory of the China Meteorological Administration 20 km to the southeast, and PM2.5concentration measured at the Beijing Olympic Center Observatory 4 km to the northeast. UTC+8 denotes Coordinated Universal Time + 8 h and represents local solar time in hours.a10-m wind speed (WS) and mixing layer height (MLH) above ground level (AGL).bLWC and relative humidity (RH);cN2O and HONO concentrations;dPM1nitrate and NO2concentrations;ePM1sulfate and SO2concentrations;fozone (O3) and ammonia (NH3) concentrations; andgblack carbon (BC) and PM2.5concentrations. The campaign sampled the tail end of a haze event on December 4, terminated by passage of a cold front on December 5 and followed by variable conditions on December 6–15 (not shown, note break in time axis). It then sampled an extended pollution episode on December 16–22 with initially moderate RH of 40–75% (Stage I), followed by high RH (>75%) including dense nighttime fog at the Beijing Observatory (Stage II), and ending on December 22 with the passage of a cold front. Nighttime periods are shaded. Sulfate and nitrate measurements are from the HR-AMS instrument with a size cut of 1-μm diameter (see text). Field observations Figure 1 shows the time series of selected variables measured at our field site on the rooftop of an Institute of Atmospheric Physics (IAP) building in urban Beijing during December 4–22, 2016. The start of the campaign on December 4 sampled the end of a haze event that terminated on December 5 with passage of a cold front. Variable conditions were observed during December 6–15 (data not shown). An extended haze event then developed over the December 16–22 period, with 24-h average PM 2.5 exceeding 200 μg m −3 for 6 successive days before a cold front swept in with clean air on December 22. Fig. 1: Chronology of a winter haze event. The figure shows the time series of meteorological parameters and chemical species measured in Beijing on December 4–22, 2016. The measurements were made from the roof of an Institute of Atmospheric Physics (IAP) building except for liquid water content (LWC) measured at the Beijing Observatory of the China Meteorological Administration 20 km to the southeast, and PM 2.5 concentration measured at the Beijing Olympic Center Observatory 4 km to the northeast. UTC+8 denotes Coordinated Universal Time + 8 h and represents local solar time in hours. a 10-m wind speed (WS) and mixing layer height (MLH) above ground level (AGL). b LWC and relative humidity (RH); c N 2 O and HONO concentrations; d PM 1 nitrate and NO 2 concentrations; e PM 1 sulfate and SO 2 concentrations; f ozone (O 3 ) and ammonia (NH 3 ) concentrations; and g black carbon (BC) and PM 2.5 concentrations. The campaign sampled the tail end of a haze event on December 4, terminated by passage of a cold front on December 5 and followed by variable conditions on December 6–15 (not shown, note break in time axis). It then sampled an extended pollution episode on December 16–22 with initially moderate RH of 40–75% (Stage I), followed by high RH (>75%) including dense nighttime fog at the Beijing Observatory (Stage II), and ending on December 22 with the passage of a cold front. Nighttime periods are shaded. Sulfate and nitrate measurements are from the HR-AMS instrument with a size cut of 1-μm diameter (see text). Full size image Wind speed during the December 16–22 haze event was persistently low in the range of 0.3–1.5 m s −1 and the mixed layer height (MLH) was less than 600 m above ground level (AGL), decreasing to 300 m at night. The early part of the event on December 16–19 (labeled Stage I in Fig. 1 ) had moderate RH in the 40–75% range. On December 20–21 (Stage II) the RH rose to above 75% as temperatures cooled to an average of 271 K at night, and dense nighttime fog with LWC as high as 0.5 g m −3 was observed at the Beijing Observatory meteorological station 20 km to the south (Fig. 1 ). Beijing International Airport also reported fog during that period (Supplementary Fig. 1 ). Dense fog was not observed at our site, but the visibility dropped below a few hundred meters and low clouds formed just 50 m above ground (Supplementary Fig. 2 ). PM 2.5 concentrations rose to over 400 μg m −3 during the high-RH period (Stage II) in concert with a rise in sulfate, while nitrate remained at the same concentration as in Stage I (47 μg m −3 ). Black carbon (BC) increased from 9.4 to 13.1 μg m −3 . SO 2 concentrations were relatively high in Stage I but nearly depleted in Stage II, indicating rapid oxidation of emitted SO 2 to sulfate. 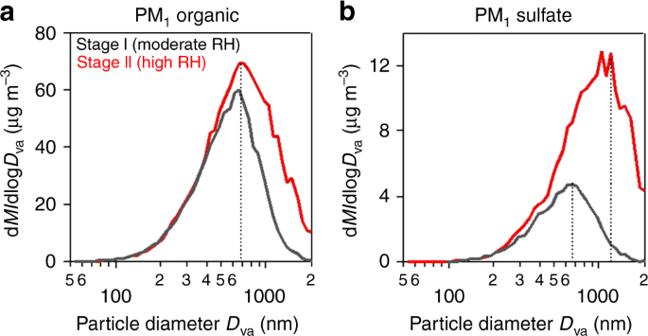Fig. 2: Size distributions of organic and sulfate particles. The Figure shows mass-based size distributions of (a) organic and (b) sulfate particles in Stages I and II of the December 16–22, 2016 haze event.Mdenotes mass andDvadenotes particle vacuum aerodynamic diameter. The measurements were made by the HR-AMS instrument with 50% size cut at 1-μm diameter, hence the data are shown as PM1(particulate matter with less than 1-μm diameter). Mass modal diameters are shown as dotted lines. Figure 2 shows that the sulfate particles measured by high-resolution aerosol mass spectrometer (HR-AMS) shifted to larger sizes during Stage II while the organic particles did not, consistent with sulfate formation taking place in fog and low cloud (cloud-mediated coagulation would have affected both sulfate and organic particles). Mean PM 2.5 increased from 210 μg m −3 in Stage I to 330 μg m −3 in Stage II, while sulfate measured by HR-AMS increased fourfold from 10 to 40 μg m −3 . The sampling efficiency of the HR-AMS instrument (PM 1 ) drops off rapidly for particles above 1-μm diameter [30] , implying that actual sulfate levels during Stage II were probably much higher than measured. Indeed, PM 2.5 sulfate concentrations measured at the site by on-line ion chromatography (URG-9000D Ambient Ion Monitor) were 1.5-2 times larger than the HR-AMS measurements during Stage II (Supplementary Fig. 3 ). Some of the sulfate particles could even be larger than PM 2.5 due to swelling at high RH. Fig. 2: Size distributions of organic and sulfate particles. The Figure shows mass-based size distributions of ( a ) organic and ( b ) sulfate particles in Stages I and II of the December 16–22, 2016 haze event. M denotes mass and D va denotes particle vacuum aerodynamic diameter. The measurements were made by the HR-AMS instrument with 50% size cut at 1-μm diameter, hence the data are shown as PM 1 (particulate matter with less than 1-μm diameter). Mass modal diameters are shown as dotted lines. Full size image Evidence for SO 2 oxidation by HONO A remarkable feature of the observations in Stage II is the large rise in N 2 O concentrations concurrently with sulfate. N 2 O is a major greenhouse gas with a globally dominant biogenic source [31] . It is chemically inert in the troposphere. Vehicles and coal combustion may be a significant source of N 2 O in Beijing [32] , but this would not explain the N 2 O rise in Stage II because no parallel rise was observed for BC (Fig. 1 ). 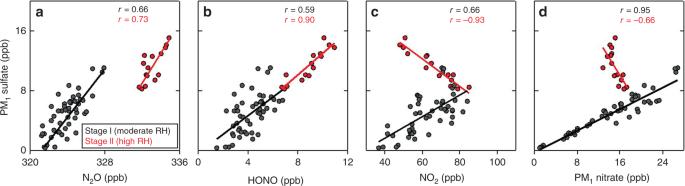Fig. 3: Relationships between sulfate and nitrogen oxide concentrations. Data are shown for Stages I and II of the December 16–22, 2016 haze event. Concentrations of sulfate and nitrogen oxides are expressed in common parts per billion (ppb) units (1 μg m−3sulfate = 0.23 ppb atT= 273.15 K). Individual points are hourly mean values from Fig.1during nighttime hours (19:00–6:00 local time). The figure shows scatterplots of PM1sulfate versusanitrous oxide (N2O);bnitrous acid (HONO);cnitrogen dioxide (NO2);dPM1nitrate. Pearson correlation coefficients (r) and reduced-major-axis regression lines are shown separately for Stages I and II. Figure 3 shows the relationships between the concentrations of sulfate and different nitrogen oxide species (N 2 O, HONO, NO 2 , and PM 1 nitrate) observed in Stages I and II. The relationships are shown only for nighttime hours (19:00–06:00) to minimize strong common dependences on diurnal changes in mixed layer depth, and to avoid the effect of fast HONO photolysis in the daytime. Sulfate correlates positively with all species in Stage I, which may reflect common dependences on atmospheric mixing and ventilation. In Stage II, sulfate is positively correlated with N 2 O (including a step increase) and with HONO, but negatively correlated with NO 2 and nitrate. This suggests a change in the regime for sulfate production in Stage II with associated production of N 2 O. Looking back at the tail end of the previous haze event on December 4, which also featured high-RH conditions, we again see elevated N 2 O together with sulfate (Fig. 1 ). Fig. 3: Relationships between sulfate and nitrogen oxide concentrations. Data are shown for Stages I and II of the December 16–22, 2016 haze event. Concentrations of sulfate and nitrogen oxides are expressed in common parts per billion (ppb) units (1 μg m −3 sulfate = 0.23 ppb at T = 273.15 K). Individual points are hourly mean values from Fig. 1 during nighttime hours (19:00–6:00 local time). The figure shows scatterplots of PM 1 sulfate versus a nitrous oxide (N 2 O); b nitrous acid (HONO); c nitrogen dioxide (NO 2 ); d PM 1 nitrate. Pearson correlation coefficients ( r ) and reduced-major-axis regression lines are shown separately for Stages I and II. Full size image N 2 O is a product of the aqueous-phase oxidation of SO 2 by HONO [28] , [29] . HONO is moderately soluble in water (Henry’s law constant K H = 49 M atm −1 at 298 K) and dissociates as a weak acid ( pK a = 3.2 at 298 K) to increase its partitioning in the aqueous phase [33] . The aqueous-phase oxidation of SO 2 by HONO can be expressed stoichiometrically as follows [28] , [29] : 
    2N(III) + 2S(IV)→N_2O↑ + 2S(VI) + other products. (R1) Here N(III) ≡ HONO(aq) + NO 2 − denotes the dissolved HONO species, S(IV) ≡ SO 2 ∙H 2 O + HSO 3 − + SO 3 2− denotes the dissolved SO 2 species, and S(VI) ≡ H 2 SO 4 (aq) + HSO 4 − + SO 4 2− denotes the sulfate species. The other products may include H 2 O or H + depending on the speciation of N(III), S(IV), and S(VI). A laboratory study by Martin et al. [28] gives a rate expression for sulfate formation from reaction (R1) at pH < 4: 
    d[ S( VI)]/dt = k_1[ H^ + ]^0.5[ N( III)][S(IV)],
 (1) where k 1 = 142 M −3/2 s −1 . Another study by Oblath et al. [27] gives a rate expression 
    d[ S( VI)]/dt = k_1^'[ H^ + ][ N( III)][S( IV],
 (2) with k' 1 = 4800 M −2 s −1 for 3 < pH < 7. Even though these rate expressions show positive [H + ] dependences, the rates actually increase with pH because both [S(IV)] and [N(III)] are inversely dependent on [H + ] over the relevant pH range. The increase of N 2 O in Stage II concomitant with sulfate suggests that reaction (R1) could be a source of sulfate. However, the slopes of the sulfate-N 2 O regression lines in Fig. 3 are similar for Stages I and II and not consistent with the 2:1 stoichiometry of reaction (R1). A possible explanation is that the PM 1 sulfate measurements underestimated total sulfate concentrations during Stage II, as shown above. In addition, it is likely that the correlations and slopes are mainly driven by mixing rather than chemistry, as is frequently observed in polluted air masses [34] , [35] . The signature of the reaction (R1) taking place in Stage II would then be manifested by the step increase in N 2 O between the two Stages. Importance of fog and cloud Reaction (R1) requires fog or cloud to proceed at an appreciable rate. LWCs in haze are too low. It also requires a relatively high pH. The mean gaseous ammonia concentration observed during Stage II was 14 ppb (Fig. 1 ), typical of previous observations during haze events [36] and mainly attributable to emissions from fuel combustion [37] . Fog has a much higher pH than haze under high-ammonia conditions because of efficient scavenging of ammonia at high LWC. Whereas ammonia volatility limits the pH of haze aqueous solutions to a 4–5 range even with ammonia in large excess [19] , [20] , [38] , [39] , [40] , the corresponding pH range in fog is 6–7 [9] , [13] , [21] , [41] , [42] . Higher pH in haze can be achieved if dust is a significant component [9] , [21] , [42] but low LWC is still a limitation. PM 2.5 concentrations of dust cations (Ca 2+ , Mg 2+ ) were low at our site, as described in the “Methods” section. Our sampling site did not actually experience fog during Stage II, but the cloud deck extended down to 50 m (Supplementary Fig. 2 ), and surface air would have been processed by that low cloud and/or by fog elsewhere. We estimate a fog/cloud pH of 5.7 on the basis of our mean measured value of 14 ppb total ammonia to be partitioned into the fogwater; a fog LWC of 0.15 g m −3 ; sulfate, nitrate, and chloride PM 2.5 present as their ammonium salts; and a temperature of 271 K (see “Methods”). Past observations for Beijing in winter indicate a fog/cloud pH range of 4.7–6.9 [7] , [11] , [26] , [43] , [44] . Sensitivity to pH will be examined in the “Discussion” section. We can estimate the e-folding lifetime for SO 2 oxidation by HONO in nighttime fog on the basis of a fog with pH 5.7 and LWC of 0.15 g m −3 , and assuming a mean nighttime total HONO concentration of 9 ppb as measured during Stage II (Fig. 1 ). This involves applying the rate expression for reaction (R1) with Henry’s law and acid dissociation constants computed at 271 K (Supplementary Table 1 ). We find a fogwater nitrite (N(III), mainly as NO 2 − ) concentration of 2.2 μmol L −1 , which leads to an e-folding SO 2 lifetime of 3.8 h using the rate expression of Martin et al. [28] extended to pH 5.7 but 79 h using the rate expression of Oblath et al. [27] . The former would imply a major role of HONO as SO 2 oxidant while the latter would imply an insignificant role. As we will see, the HONO concentration in fog could actually be much higher than measured at our site, which would increase the importance of reaction (R1). The observed increase of N 2 O in Stage II does suggest an important role for reaction (R1). Evidence for SO 2 oxidation by NO 2 and production of HONO A remarkable result in Fig. 3 is the positive correlation of sulfate with HONO during Stage II, and the negative correlations with NO 2 and nitrate. Aqueous-phase loss of NO 2 during haze and fog is generally thought to be driven by particle-phase disproportionation to HONO and HNO 3 [11] , but if this were the case we would expect an increase in nitrate during Stage II in contrast to what was observed (Figs. 1 and 3 ). Aqueous-phase oxidation of S(IV) by NO 2 (aq) in fog is an alternative explanation for the depletion of NO 2 and produces both HONO and sulfate [28] , which would be consistent with the positive correlation observed between the two (Fig. 3 ): 
    S( IV) + 2NO_2( aq) + H_2O→S( VI) + 2H^ + + 2NO_2^ -. (R2) Laboratory studies give a rate expression for reaction (R2) as 
    d[ S( VI)]/dt = k_2[NO_2( aq)][S(IV)],
 (3) with k 2 = 2 × 10 6 M −1 s −1 for the pH range 5.8–6.4 (Lee and Schwartz [45] ) and k 2 = 1.2–1.5 × 10 7 M −1 s −1 for the pH range 5.3–6.8 (Clifton et al. [46] ). For a mean nighttime NO 2 concentration of 50 ppb during Stage II (Fig. 1 ), and a fog with LWC = 0.15 g m −3 and pH = 5.7, we find an SO 2 e-folding lifetime of 1–7 min against loss by reaction (R2) depending on which value of k 2 is used, sufficiently short in any case for SO 2 depletion. Reaction (R2) further produces N(III) as \({\mathrm{NO}}_2^ -\) , which in a fog of pH 5.7 would remain in the aqueous phase and may thus go on to oxidize SO 2 by reaction (R1). If reaction (R1) is sufficiently fast, following the rate expression of Martin et al. [28] , then a steady state would be established at night between production of \({{\mathrm{NO}}_2^ -}\) in the fog by reaction (R2) and loss by reaction (R1), resulting in an effective sulfate mass yield of 2 from reaction (R2). An SO 2 oxidation mechanism in nighttime fog involving reaction (R2) followed by reaction (R1) would be consistent with our observed enhancement of N 2 O. In that mechanism, one mole of N 2 O is produced for every three moles of SO 2 oxidized. Starting from a SO 2 level of 20 ppb in Stage I (Fig. 1 ), complete oxidation of that SO 2 to sulfate would produce 7  ppb N 2 O, consistent with the ≈5 ppb increase of N 2 O observed between Stage I and Stage II (Fig. 3 ). The mechanism both produces and consumes HONO in the oxidation of SO 2 , whereas N 2 O is a terminal product, which may explain why HONO shows a positive correlation with sulfate in Stage II but not a step increase. One would similarly expect one mole of NO 2 to be consumed for every 0.5–1.5 mole of SO 2 oxidized, depending on whether oxidation by (R2) is followed by (R1). The sulfate-NO 2 slope in Fig. 3 is only −0.2 mol mol −1 , which could suggest additional NO 2 sinks associated with fog, an underestimate of sulfate in the Stage II observations as previously discussed, or a dominance of atmospheric mixing in determining the slope. 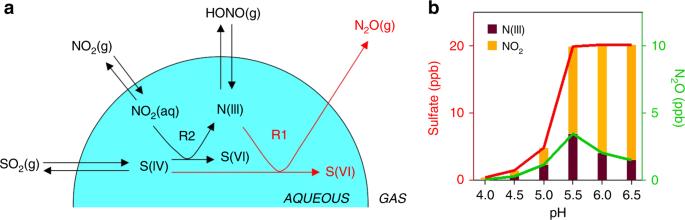Fig. 4: SO2oxidation mechanism. aIllustration of the mechanism for SO2oxidation to sulfate by NO2and HONO in fog and cloud. Here S(IV) ≡ SO2∙H20 + HSO3−+  SO32−denotes the different forms of dissolved SO2, S(VI) ≡ H2SO4(aq) + HSO4−+ SO42−denotes the different forms of sulfate, and N(III) ≡ HNO2(aq) + NO2−denotes the different forms of dissolved HONO. S(IV) is oxidized in the aqueous phase by dissolved NO2(reaction (R2)), producing N(III) which may oxidize additional S(IV) and produce N2O by reaction (R1).bpH-dependent sulfate and N2O production from the (R2) + (R1) mechanism. The plot shows accumulated concentrations of sulfate and N2O after 5 h in a nighttime fog air parcel simulation initialized with [SO2] = 20 ppb, [NO2] = 80 ppb, and [HONO] = 5 ppb, with a fog LWC = 0.15 g m−3andT= 271 K. Contributions from aqueous-phase SO2oxidation by HONO (reaction (R1)) and NO2(reaction (R2)) are shown separately. A sulfate production of 20 ppb implies complete oxidation of SO2over the 5 h. Figure 4a illustrates our proposed mechanism for sulfate formation involving reactions (R1) and (R2) in nighttime fog and cloud associated with winter haze events. We conducted air parcel model calculations to study the pH dependence of sulfate formation in this mechanism. For reaction (R1) we used the rate expression from Martin et al. [28] , because the much slower rate expression of Oblath et al. [27] would not explain the observed N 2 O enhancement. For reaction (R2) we followed the rate constant ( k 2 ) estimates of Lee and Schwartz [45] as 1.4 × 10 5 M −1 s −1 for pH < 5 and 2 × 10 6 M −1 s −1 for pH > 6, with linear interpolation between these two pH ranges. Henry’s law and acid dissociation equilibrium constants for SO 2 , NO 2 , and HONO are in Supplementary Table 1 . The air parcel was initialized with concentrations taken from the field observations during Stage I including [SO 2 ] = 20 ppb, [NO 2 ] = 80 ppb, [HONO] = 5 ppb, and then allowed to evolve as a closed system for 5 h in a nighttime fog with LWC = 0.15 g m −3 and T = 271 K. The time scale for equilibration between the gas and aqueous phases in fog is less than a few minutes [47] , so that Henry’s law can be applied to all three gases. In the case of HONO, N(III) has a lifetime against oxidation of S(IV) of 1.5 h for 20 ppb SO 2 and pH = 5.7, and this lifetime becomes longer as SO 2 is depleted. Fig. 4: SO 2 oxidation mechanism. a Illustration of the mechanism for SO 2 oxidation to sulfate by NO 2 and HONO in fog and cloud. Here S(IV) ≡ SO 2 ∙H20 + HSO 3 − +  SO 3 2− denotes the different forms of dissolved SO 2 , S(VI) ≡ H 2 SO 4 (aq) + HSO 4 − + SO 4 2− denotes the different forms of sulfate, and N(III) ≡ HNO 2 (aq) + NO 2 − denotes the different forms of dissolved HONO. S(IV) is oxidized in the aqueous phase by dissolved NO 2 (reaction (R2)), producing N(III) which may oxidize additional S(IV) and produce N 2 O by reaction (R1). b pH-dependent sulfate and N 2 O production from the (R2) + (R1) mechanism. The plot shows accumulated concentrations of sulfate and N 2 O after 5 h in a nighttime fog air parcel simulation initialized with [SO 2 ] = 20 ppb, [NO 2 ] = 80 ppb, and [HONO] = 5 ppb, with a fog LWC = 0.15 g m −3 and T = 271 K. Contributions from aqueous-phase SO 2 oxidation by HONO (reaction (R1)) and NO 2 (reaction (R2)) are shown separately. A sulfate production of 20 ppb implies complete oxidation of SO 2 over the 5 h. Full size image As shown in Fig. 4b , we find in this air parcel model that reactions (R1) and (R2) are sufficiently fast for complete conversion of SO 2 to sulfate at pH > 5.5, with a maximum contribution from reaction (R1) at pH 5.5. At higher pH, the faster kinetics of reaction (R2) decrease the role of reaction (R1) in competing for SO 2 oxidation, resulting in a lower yield of N 2 O. The N 2 O yield would also be low (<2 ppb) if we used the faster kinetics for (R2) from Clifton et al. [46] . The observed N 2 O enhancement of ≈5 ppb is most consistent with the kinetics of Lee and Schwartz [45] for (R2) and Martin et al. [28] for (R1), with a fog/cloud pH of 5.5 (Fig. 4b ), but uncertainties are obviously large. Further analysis will require better kinetic information for reactions (R1) and (R2). Decreasing ammonia emissions to bring cloud pH below 5 would shut down the mechanism (Fig. 4b ), but other SO 2 oxidation pathways may then take over such as TMI-catalyzed autoxidation [22] . The role of (R2) + (R1) as a source of HONO and N 2 O is of interest, considering that HONO photolysis is a major source of radicals during winter haze [48] and that N 2 O is a major anthropogenic greenhouse gas. Previous studies have found that HONO in Beijing haze has a large source from direct vehicular emissions [48] , [49] and this could explain the rise of HONO observed during Stage I (Fig. 1 ). However, the doubling of HONO concentrations from Stage I to Stage II suggests that (R2) could be an important source of HONO during haze events. With regard to N 2 O, the most relevant comparison is to the national anthropogenic source for China, estimated to be 2141 Gg a −1 with a dominant contribution from agriculture [50] . For a rough estimate, let us assume that (R2) + (R1) is the dominant SO 2 sink during high-RH winter haze, accounting for ~8% of winter days (data downloaded from https://rp5.ru/ ), and that the N 2 O molar yield is 20% based on the upper limit (pH 5.5) of Fig. 4b . The Multi-resolution Emission Inventory for China estimates a national SO 2 emission of 13.4 Tg a −1 in 2016 [51] , which would then imply a corresponding N 2 O source of 36.8 Gg a −1 . This is small compared with the national inventory total, but not negligible as a component of N 2 O emission from the energy sector estimated to be 232.7 Gg a −1 in 2012 [50] . In summary, we have shown from field observations of an extended winter haze PM 2.5 pollution event in Beijing that aqueous-phase oxidation of SO 2 by NO 2 and HONO in nighttime fog and low cloud provides a plausible mechanism for explaining the rapid production of sulfate PM 2.5 . Production of sulfate in fog and cloud is consistent with the observed shift in the sulfate size distribution to larger sizes. High-RH conditions with widespread fog and low cloud formation are typical of severe winter haze events in Beijing [2] , [26] . This provides high LWCs for aqueous-phase reactions to occur, together with high pH (>5.5) from efficient uptake of ammonia. Based on available aqueous-phase kinetic data, such high-LWC high-pH conditions should allow fast oxidation of SO 2 by NO 2 to produce HONO, and subsequent fast oxidation of SO 2 by HONO to produce N 2 O. There remains large uncertainty in these kinetic data. But such a mechanism is consistent with our field observations of N 2 O enhancement, HONO enhancement, NO 2 depletion, and near-complete SO 2 depletion concurrent with fast sulfate production as RH increased during the haze event. Further work should target better understanding of the laboratory kinetics and products of the aqueous-phase reactions of SO 2 with NO 2 and HONO. Field campaign The field campaign was conducted at the Tower Site of the IAP, Chinese Academy of Science (39°58′N, 116°22′E) in Beijing, China from 4 to 22 December of 2016. This site is located around the 3rd ring road of north Beijing, surrounded by residential infrastructure and an arterial road to the east (360 m). Measurements were made from a rooftop laboratory 8 m above ground and with no interference from neighboring buildings. All data presented in this paper were hourly averaged (local time, UTC+8). A HR-AMS was deployed during the field campaign to obtain chemical composition and size distributions of non-refractory particulate matter smaller than 1-μm diameter (NR-PM 1 ). A shared PM 2.5 cyclone inlet (Model URG-2000-30ED) and a diffusion dryer were used prior to the sampling. Detailed information on the operation of HR-AMS during the sampling campaign can be found in previous literature [4] , [52] . Additional measurements of aerosol composition were made with a URG-9000D Ambient Ion Monitor for water-soluble ions including a BGI-VSCC PM 2.5 cyclone upstream. Anion analysis was performed using the IonPac AS19 hydroxide-selective anion-exchange column, which can effectively separate sulfate from HMS. PM 2.5 mass concentration was measured by a TDMS-TEOM PM 2.5 analyzer (Thermo Fisher Scientific, Model 1405) at the Beijing Olympic Center Observatory, which is 4 km to the northeast of the sampling site. Fog LWC was measured by a TP/W VP-3000 ground-based 12-channel microwave radiometer (Radiometrics Corp.) at the Beijing Observatory of the China Meteorological Administration (CMA), 20 km to the south of our sampling site. Gaseous and meteorological data were also collected at the site. An Aerodyne high-resolution time-of-flight chemical ionization mass spectrometer measured HONO concentrations [53] . N 2 O concentration was measured with a real-time CH 4 /N 2 O Analyzer (Los Gatos Research, Inc.). Concentrations of O 3 , SO 2 (precision 0.5 ppb), and NO 2 were measured with Thermo Fisher Scientific instruments (Models 49 i , 43 i , 42 C ), and NH 3 by a Los Gatos Research analyzer. Vertical profiles of meteorological parameters, including wind speed and direction, temperature, and RH were measured from the IAP 325-m meteorological tower. Figure 1 shows the time series of fog LWC measured at the Beijing CMA Observatory, 20 km to the south of our IAP sampling site. No fog was observed at the Observatory during Stage I (December 16–19) but pervasive nighttime fog was observed during Stage II (December 20–21) with a mean LWC of 0.15 g m −3 and maximum of 0.4 g m −3 . CMA forecasts advised for strong fog (visibility 50–200 m) and extra-strong fog (visibility <50 m) across the North China Plain during the Stage II period ( http://products.weather.com.cn/product/Index/index/procode/YB_W_24.shtml ). Previous studies have reported fog LWCs of 0.2–0.3 g m −3 in the North China Plain in association with winter haze events [54] , [55] . Calculation of fog/cloud pH We estimated fog/cloud pH values during Stage II by assuming a pre-fog atmosphere with the mean composition observed at the IAP field site, and adding to that atmosphere an LWC of 0.15 g m −3 . The IAP field site did not experience fog during Stage II, but cooling of a few degrees would have caused fog to form (as apparent in the low clouds observed 50 m above the site, Supplementary Fig. 2 ) and drive partitioning of gases into the aqueous phase. We can then estimate the fog/cloud pH from the partitioning of the relevant chemicals initially present in pre-fog air as defined by the mean conditions of Stage II (Fig. 1 ). This includes 14 ppb NH 3, 2 ppb SO 2 , and PM 2.5 with electroneutral composition [SO 4 2− ] = 3 × 10 −3 mol L −1 , [NO 3 − ] = 6 × 10 −3 mol L −1 , [Cl − ] = 1 × 10 −3 mol L −1 , and [NH 4 + ] = 1.3 × 10 −2 mol L −1 . We also include 400 ppm CO 2 , and neglect organic acids which are low under winter haze conditions [56] . Alkaline dust would increase the pH and is found to be important in precipitation data for winter Beijing [14] , [57] but our mean Stage II PM 2.5 measurements show [Ca 2+ ] = 1.2 × 10 −5 mol L −1 and [Mg 2+ ] = 2.1 × 10 −5 mol L −1 for the principal crustal cations, negligible relative to [NH 4 + ]. Thus we ignore the contribution of dust in the pH calculation, acknowledging that this may cause an underestimate of pH since dust could be present in larger particle sizes. We performed the pH calculation for a temperature of 271 K with the Henry’s law and acid dissociation constants in Supplementary Table 1 . We obtain in this manner a fog/cloud pH of 5.7.